Evolution of oil droplets in a chemorobotic platform Evolution, once the preserve of biology, has been widely emulated in software, while physically embodied systems that can evolve have been limited to electronic and robotic devices and have never been artificially implemented in populations of physically interacting chemical entities. Herein we present a liquid-handling robot built with the aim of investigating the properties of oil droplets as a function of composition via an automated evolutionary process. The robot makes the droplets by mixing four different compounds in different ratios and placing them in a Petri dish after which they are recorded using a camera and the behaviour of the droplets analysed using image recognition software to give a fitness value. In separate experiments, the fitness function discriminates based on movement, division and vibration over 21 cycles, giving successive fitness increases. Analysis and theoretical modelling of the data yields fitness landscapes analogous to the genotype–phenotype correlations found in biological evolution. Evolution has been widely studied as a the source of adaptation and complexity in biology [1] , and as such has more recently been emulated in artificial intelligence as evolutionary optimization algorithms used to evolve electronic circuits [2] , [3] . However, these experiments in embodied evolution have been limited to engineering and robotics, and the embodied evolution of populations of physically interacting individuals has not yet been explored [4] . There has been recent interest in the development of chemical systems, showing complex behaviours [5] from simple input recipes, as potential minimal models for exploring the interface between robotics [6] , [7] , artificial intelligence [8] , nonlinear chemical systems and evolutionary dynamics. This is because biological evolution, a process that relies on populations of replicating individuals who have the ability to inherit, exhibit variation and undergo selection by the environment over successive generations, has been able to create extremely complex and sophisticated biological systems [1] . We therefore hypothesized that the construction of a robot capable of producing well-defined chemical formulations presented as discrete physical objects, in this case oil droplets, could be used as a platform to drive the evolution of populations of the oil droplets [9] . Such a platform would not only require a robot to produce and mix the chemical formulations but also to produce the objects as oil droplets in a dish [4] , and this would be driven by a software programme [10] , [11] . The droplets would then be observed by a sensor system, here a video camera, and then the droplet compositions varied using an evolutionary algorithm that could develop the desired properties of the droplets against a well-defined desired test, see Fig. 1 . 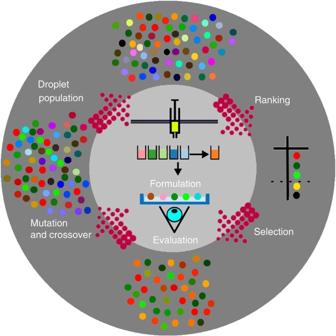Figure 1: Schematic describing the evolutionary process. The inner circle represents a zoomed part of the robotic process and outer circle represents the computational algorithm. In the first step a random selection of the droplet formulations is used as the starting ‘Droplet Population’ and this forms the experimental formulations. These droplets are generated in the ‘Formulation’ step and are placed into a Petri dish. The droplet behaviours are then recorded using a camera and then image analysis is conducted against a user-desired property (for example, colour) in the ‘Evaluation’ step. The droplets are ranked in terms of desired property automatically, and the least good rejected in the ‘Ranking’ step allowing a new population to be ‘Selected’. Meanwhile, the accepted formulations are used as a basis to create a new ‘Droplet Population’ after random ‘Mutation’ and ‘Crossover’. This process continues for 21 cycles and the fitness is recorded. Figure 1: Schematic describing the evolutionary process. The inner circle represents a zoomed part of the robotic process and outer circle represents the computational algorithm. In the first step a random selection of the droplet formulations is used as the starting ‘Droplet Population’ and this forms the experimental formulations. These droplets are generated in the ‘Formulation’ step and are placed into a Petri dish. The droplet behaviours are then recorded using a camera and then image analysis is conducted against a user-desired property (for example, colour) in the ‘Evaluation’ step. The droplets are ranked in terms of desired property automatically, and the least good rejected in the ‘Ranking’ step allowing a new population to be ‘Selected’. Meanwhile, the accepted formulations are used as a basis to create a new ‘Droplet Population’ after random ‘Mutation’ and ‘Crossover’. This process continues for 21 cycles and the fitness is recorded. Full size image The reason we are interested in formulating oil-droplet formulations using a robotic system was to see whether we could achieve the robot-driven evolution of these oil droplets [12] , and over multiple successive generations observe correlations between droplet behaviour and composition analogous to genotype–phenotype correlations from analogous biological experiments [13] . Such simple oil droplets could be used as models for primitive protocells [14] since they are characterized by an interface (for example, oil–water) or membrane separating the inside and the outside of the cell; yet they are so primitive that they had been considered to lack genetic material. However, theoretical simulations using the Graded Autocatalysis Replication Domain model clearly suggest that formulations or ‘composomes’, such as those proposed here, could be evolvable [15] . This approach therefore paves the way for exploring complex chemical systems by embodied evolution, as well as a better understanding of the minimal infrastructure required for the evolution of chemistry outside of biology [6] . The process of assisting the evolution via the robot [4] , [6] is itself important since the automation will allow us to do many comparisons, as well as a large number of experiments under well-controlled conditions. In addition, by varying the input ‘compositions’ it is hypothesized that emergent behaviour will result from this coupling [7] , [8] , such as that seen in soft robotics whereby morphology and topology have been combined [16] . Indeed, the development of hybrid chemorobotic systems capable of combinatorial oil-droplet formation, as well as assisting the process of evolution, has not been possible because of many hardware and software constraints. These requirements include the need to develop a fluid-handling robotic system with autonomous control, sensing the ability to reliably generate a large population of droplets, as well as the automation of the oil-droplet formation–evaluation–cleaning cycle. In addition, solving these issues is also of potential benefit in other areas such as the emerging field of systems chemistry, which seeks to understand and explore the complex chemical systems, networks and emergent behaviours that arise from very simple inputs [5] . In our work we have developed a novel means of exploring complex chemical systems by controlling the interface between robotics, artificial intelligence, complex chemical systems and evolutionary dynamics. Self-propelled oil droplets have long been studied as primitive chemical machines, transferring chemical energy to kinetic energy [17] . The key mechanism for the motion of oil droplets in aqueous media is the Marangoni effect, an asymmetry of interfacial surface tension around the droplet [18] . Small inhomogeneities in the surface of the aqueous phase cause the droplet to no longer be completely symmetrical, meaning that the surface tensions around the droplet become unbalanced and the droplet is pulled in a certain direction. Certain oils, such as 1-pentanol form droplets on the surface of an aqueous phase but dissolve at a rate dictated by their aqueous solubility [19] . This results in an increase in concentration of the oil in the aqueous phase close to the droplet, and therefore a decrease in interfacial tension at the trailing edge of a moving droplet. This surface tension gradient is responsible for rapid movement and deformation, which sometimes splits the droplet apart. A chemical reaction such as deprotonation of a carboxylic acid to produce an anionic surfactant may result in asymmetric accumulation of the surfactant product at the oil–water interface, further contributing to the asymmetry of surface tension [20] . In our work we develop a means of exploring complex chemical systems by controlling the interface between robotics, artificial intelligence, complex chemical systems and evolutionary dynamics. Evolvable oil-droplet system For our evolvable droplet system we chose four components, whose relative quantities form our compositional genome: 1-Octanol, Diethyl phthalate, 1-Pentanol and either octanoic acid or dodecane as the fourth ingredient, aiming for droplets that have motility, ability to divide [21] , stability and a range of solubilities, densities and viscosities, see Fig. 2 . In this way, the droplets of oil in water provide a chemical compartment with characteristics that depend on the density of the droplet, the interfacial tension between aqueous and organic phases, the polarity of the oil and any reactions that occur at the interface. 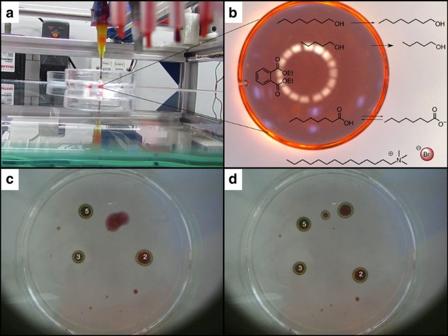Figure 2: Droplets as placed and observed by the robot. (a) Side-on view of a droplet being placed by the syringe into the aqueous phase. (b) Microscope image of a typical droplet showing the chemical components of the system. Arrows show the partitioning into the aqueous phase of the oils, the larger arrow for 1-pentanol denotes far greater aqueous solubility than that for 1-octanol. (c) Droplets being tracked by the image analysis software, one of the droplets is undergoing division and its distorted shape is not recognized as circular by the software. (d) Image of the daughter droplets from the fission of the distorted droplet fromcbeing recognized by the image analysis software. Figure 2: Droplets as placed and observed by the robot. ( a ) Side-on view of a droplet being placed by the syringe into the aqueous phase. ( b ) Microscope image of a typical droplet showing the chemical components of the system. Arrows show the partitioning into the aqueous phase of the oils, the larger arrow for 1-pentanol denotes far greater aqueous solubility than that for 1-octanol. ( c ) Droplets being tracked by the image analysis software, one of the droplets is undergoing division and its distorted shape is not recognized as circular by the software. ( d ) Image of the daughter droplets from the fission of the distorted droplet from c being recognized by the image analysis software. Full size image It follows that, from just a few inputs, a wide variety of droplet behaviours emerge, allowing us to explore the potential for the discovery of emergent properties, complex behaviours and the ability to embody evolution within the compositional formulations of the oil-droplet system. Our initial trial experiments in this chemical space led to the discovery that oil droplets comprises 1-octanol, when placed in an aqueous surfactant solution at pH 13, undergo rapid movement and binary fission even though 1-octanol is not appreciably deprotonated at this pH. It would appear that 1-pentanol, being less hydrophobic, dissolves in the aqueous phase more readily, resulting in more rapid and less controlled fission. On the other hand, diethyl phthalate (DEP) is only slightly soluble in water, stable to hydrolysis and denser than water, forming well-defined rounded droplets that hang just below the surface [22] . In contrast, dodecane is less dense than water and very hydrophobic, forming irregular droplets that float on the surface. Octanoic acid is deprotonated in alkaline media, leading to the formation of an anionic surfactant, able to drive phenomena such as movement or increases in surface area. Together, these oils occupy a large range of densities, polarities and interfacial tensions, resulting in a parameter space suitable, in size and scope, for exploration as potential protocell models. One of the reasons for choosing formulations is that the chemical stability of the system should result in physical effects rather than chemical reactions, for example, hydrolysis or condensation. To explore the dynamics and assist the evolvability of the chosen oil-droplet ‘protocell’ model system, a fully automated liquid-handling robot capable of placing multiple droplets on the surface of a Petri dish of aqueous medium was constructed, equipped with a camera for video recording/image analysis and programmed using an evolutionary algorithm, see Fig. 3 and Supplementary Methods . 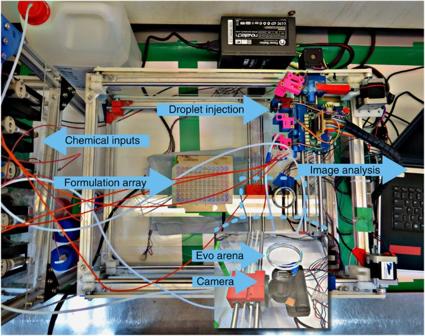Figure 3: Plan view of the robotic system. Photograph showing the pumps: cleaning and oil phases, the mixing array, the syringe array held in the X–Y stage, the evolutionary arena, the optical imaging system held below the evolution arena, the motors controlling the X–Y carriage and the computer interface. SeeSupplementary Movie 1for operation of the robot. SeeSupplementary Fig. 1for a different angle. Figure 3: Plan view of the robotic system. Photograph showing the pumps: cleaning and oil phases, the mixing array, the syringe array held in the X–Y stage, the evolutionary arena, the optical imaging system held below the evolution arena, the motors controlling the X–Y carriage and the computer interface. See Supplementary Movie 1 for operation of the robot. See Supplementary Fig. 1 for a different angle. Full size image Robotics set-up Our hybrid chemorobotic system was designed and built using rapid prototyping techniques and based upon the open source ‘RepRap’ three-dimensional (3D) printer [23] , [24] , where the extruder was replaced by a liquid-handling carriage and the software adapted for these new capabilities (see Supplementary Methods ). It is important to note that the mechanical modifications were prototyped using a RepRap 3D printer itself to manufacture the redesigned pieces, allowing for an iterative hardware development, where new versions of the modular robotic system were drafted, printed and tested. This resulted in a fully automated, highly customisable robotic platform with four input chemicals, a series of pumps, well-plate array for mixing of the chemicals and an array of syringes on a robotic stage. Further, the modularity (and iterative design philosophy) means that the robot can be readily configured for a variety of chemical, material and formulation-based studies. In our experiments, four 5-μl droplets were placed on top of the aqueous phase and a video of the resulting droplet behaviour recorded from beneath the dish using a camera at a resolution of 640 × 480 pixels at 60 fps. The X–Y carriage of the robot carries four nozzles ( Supplementary Figs 2 and 3 ), which are connected to syringe pumps to produce the reagent mixtures for the droplets in a single well of a 96-well plate ( Supplementary Fig. 4 ). Each well is stirred with a magnetic stirrer bar and the samples are prepared, before being withdrawn by an automated syringe assembly ( Supplementary Fig. 5 ). The formulations are then transferred to produce populations by releasing the droplets from the syringe into the aqueous phase (20 mM aqueous tetradecyltrimethylammonium bromide (TTAB), pH 13.00). A fifth nozzle is used to add the aqueous phase into a Petri dish that acts as the experimental arena. A cleaning nozzle is also present on the carriage, allowing for automatic cleaning (see Supplementary Fig. 6 ). After the experiment, the entire contents of the dish are automatically removed and the dish is cleaned with three washes of acetone followed by three washes of aqueous phase. During the acetone wash, the syringe is also cleaned with acetone. Lattice search To explore the emergent dynamics of the system, an evenly spaced combinatorial ‘lattice search’ was conducted over the four-chemical search space (see Supplementary Fig. 15 ), whereby the chemical formulations were composed as 8-bit entities, with 2 bits assigned to each of the relative quantities of dodecane, pentanol, octanol and DEP. Under this regime, a total of 225 unique combinations were possible (NB: as, for example, 1,1,1,1 is exactly the same as 2,2,2,2 and 0,0,0,0 is not a valid formula). After mixing, the formulations were placed into a Petri dish containing the aqueous phase to form droplets, and a 1-min video was captured twice for each formulation. During this process, we discovered and characterized a total of nine distinct behaviours, as described in Fig. 4 and Supplementary Movie 2 , displaying a great deal of complex, unexpected emergent behaviours. 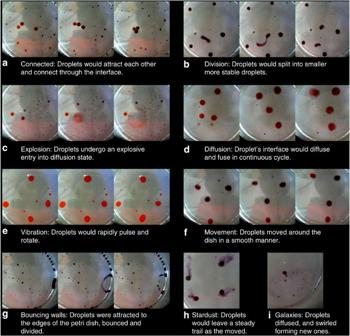Figure 4: Variety of behaviours observed in lattice search. Photographs of the droplet behaviour as a function of time (from left to right) for all the traits (given ina–i) except the ‘stardust’ and ‘galaxies’ where just one image is shown. SeeSupplementary Movie 2. Figure 4: Variety of behaviours observed in lattice search. Photographs of the droplet behaviour as a function of time (from left to right) for all the traits (given in a – i ) except the ‘stardust’ and ‘galaxies’ where just one image is shown. See Supplementary Movie 2 . Full size image This system is highly sensitive to the physical properties of the droplet, for example, aqueous solubility, surface tension, density and viscosity. The driving force for the different behaviours is related to the delicate balance between the internal forces within the droplets driven by instabilities such as the Marangoni instability, by the phase separation of the different organic components and by their residual solubility. To explore the possibility of evolving oil droplets as protocell models for different traits, behaviours or fitness, a subsequent series of experiments employing an evolutionary programming approach within our robotic platform was undertaken. The algorithm was set up with point mutation and two-parent recombination, using roulette selection, both to select parents for each subsequent generation and to cull ‘dead’ individuals (See Supplementary Table 1 for more details). Each set of inputs consisted of four real numbers, which were constrained to sum to one, and which scaled with an 8-bit resolution. Each of these numbers directly corresponded to the relative quantity of one of the substances used in the formulations for each optimization. Evolutionary experiments Three fitness functions were explored separately using the evolutionary algorithm, all of which were imposed on the basis of the analysis of 1 min of video taken after the introduction of exactly four droplets to the aqueous phase: the division fitness function describes the number of droplets above a predefined threshold, counted 1 min after the introduction of the droplets; the movement fitness function describes the average velocity of the droplets throughout the experiment (in pixels per frame), the vibration fitness function evaluates the angular velocity in degrees per frame. These fitness functions are described in detail in Supplementary Methods ). Each fitness function was applied to three repeats of a genome with the minimum between the mean and the median being taken as the final fitness of that individual. Each full evolutionary experiment was carried out over 21 generations and repeated three times in total, see Supplementary Movies 3–5 . Over 21 generations the fitness values showed significant statistical values (F div =104.1, F mot =75.9, F vib =43.6 and p<10 −8 for all the fitness values, by analysis of variance (ANOVA) test between first and last generations; this is a standard statistical test for this type of data see Supplementary Methods for more details). We were thus able to show that the oil-droplet composition could be evolved to give a series of different traits or behaviours, see Fig. 5 . It is also worth noting, from a combinatorial point of view, that the number of discrete experiments defined by the input parameters is ca. 1.678 × 10 7 experiments (24 bit); therefore, an exhaustive search for all possible ingredient ratios (at 6 mins per experiment), without the evolutionary algorithm, would have taken 6 × 10 9 s or 575 years, rather than 2 weeks per fitness (that is, the state space was searched in <0.5% of the combinatorial time). In the next step, the individual input–output pairs from the evolutionary programme were modelled (see Supplementary Methods for details) to produce a fitness diagram. 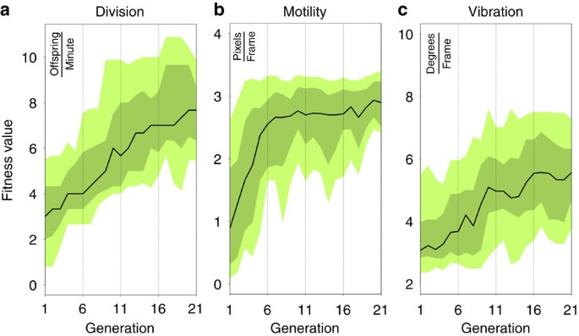Figure 5: Fitness increase over successive generations. Graphs showing the change in fitness (evolutionary trajectory) over each successive generation of experiments for (a) division, (b) motion and (c) vibration. For each of the three behaviours each set of experiments was repeated three times. The black line corresponds to the median for each generation and the dark-green bounds the distribution between the upper and lower 25th percentile and the light-green bounds between the upper and lower 10th percentile. Figure 5: Fitness increase over successive generations. Graphs showing the change in fitness (evolutionary trajectory) over each successive generation of experiments for ( a ) division, ( b ) motion and ( c ) vibration. For each of the three behaviours each set of experiments was repeated three times. The black line corresponds to the median for each generation and the dark-green bounds the distribution between the upper and lower 25th percentile and the light-green bounds between the upper and lower 10th percentile. Full size image Fitness landscapes The model was then used to estimate the fitness at each location, allowing the construction of a ternary fitness map, see Fig. 6 and Supplementary Methods . The maps show a diversity in response to the variation in individual chemical components, whereby the variation in one chemical component (for example, Octanol and DEP) can have an effect on multiple characteristics (for example, division and motility). The fitness landscapes were produced through a multistep analytical pipeline. The results from the GA were first collated and passed through a radial basis function kernel ridge regression to produce a quadratic model (that is, including direct effects of constituents and also two-way interactions between them). This model was then queried through a grid search (three parameters at a time, with the fourth fixed as zero) to estimate the fitness across the entire range of possibilities. In addition, the nonlinear response of the landscapes, and particularly the multiple optima within the division and vibration landscapes, are sufficient to demonstrate that mutations in the chemical input formula can have separate effects from the individual effects of the constituent mutations. 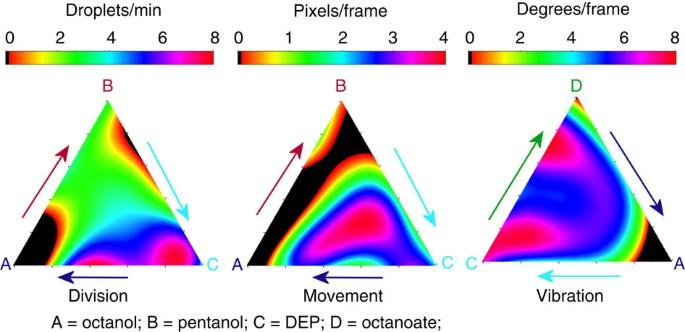Figure 6: Fitness landscapes for each fitness function. Section of the ternary Fitness maps derived from the experimental data for division, motion and vibration. For each of these maps the variation of volume fraction of three of the four components is plotted (with the fourth parameter held constant at zero) with the fitness values (red highest, black the lowest). This means that, for a given fitness, the volume fractions of the three components varied can be read off. Multiple fitness peaks were observed in the experimental data set and using this map it is possible to read off the best volume fractions of the input chemicals to achieve the best behaviours. SeeSupplementary Figs 12 and 13for more details. Figure 6: Fitness landscapes for each fitness function. Section of the ternary Fitness maps derived from the experimental data for division, motion and vibration. For each of these maps the variation of volume fraction of three of the four components is plotted (with the fourth parameter held constant at zero) with the fitness values (red highest, black the lowest). This means that, for a given fitness, the volume fractions of the three components varied can be read off. Multiple fitness peaks were observed in the experimental data set and using this map it is possible to read off the best volume fractions of the input chemicals to achieve the best behaviours. See Supplementary Figs 12 and 13 for more details. Full size image Both division and movement show their optima in the octanoic-free plane; this substance has purely negative effects on these behaviours. However, some octanoic acid is required for optimal response in the vibration landscape. In both the division and the vibration landscape, dual optima with low enough difference to be considered equivalently fit are found. Populations on these landscapes have been observed to evolve to one peak or the other; coexistence is selected against, as hybrid ‘children’ prove weaker than either individual parent. Taken together, these results show that even simple four-chemical oil-droplet formulations result in complex landscapes. This demonstrates a proof of principle for the concept of robotically assisted evolution of simple chemical systems. By using a robotic assistant as the key automating component to facilitate the evolutionary process we are able to demonstrate that the system evolves as whole. This means that it is the robotic system that allows us to explore the potential to evolve an oil droplet as a protocell model for a particular task, such as splitting, then seeking out other droplets and fusing with them (see Supplementary Movie 6 ), allowing the chemicals within to mix and react. In the current system we have predefined fitness functions but another important point will be to explore ‘novelty’, that is, the emergence of unexpected features, functions or behaviours, and to also show that the co-evolution of these features could be possible. One important aspect is the ability of the user to reproduce the behaviours manually and to demonstrate robustness. To do this we set up an experiment to see whether this was possible, and indeed we were able to show that the droplets were able to coexist and exhibited the evolved behaviour together, see Fig. 6 and video Supplementary Movie 7 . 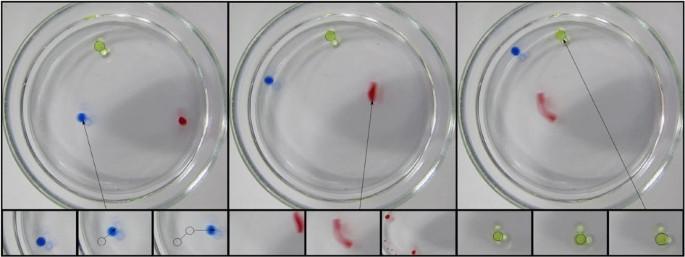Figure 7: Coexistence of evolved droplet formulations. Manual reproduction and coexistence of three highly evolved droplet formulations introduced by a user, but optimized with the robot. Each set of the three boxes focusses on the time lapse behaviour of a given trait. Colour code for the traits: blue—movement; red—division; yellow—vibration. The formulations used were (percentages octanoic acid, 1-pentanol, 1-octanol, DEP): Vibration (15.6, 8.4, 2.3 and 73.7), movement (13.6, 20.4, 45.1 and 20.9) and division (4.0, 17.9, 35.7 and 42.4). Figure 7 shows how, in a ‘control’ experiment, we took the highest fitness value oil-droplet formulations from each of the division, vibration and movement evolution experiments and manually added a droplet showing each behaviour into a single Petri dish. This demonstrates the robustness of the evolved entities to an altered environment, and also may allow the development of oil droplets as viable protocell models with desired properties for well-defined applications. Figure 7: Coexistence of evolved droplet formulations. Manual reproduction and coexistence of three highly evolved droplet formulations introduced by a user, but optimized with the robot. Each set of the three boxes focusses on the time lapse behaviour of a given trait. Colour code for the traits: blue—movement; red—division; yellow—vibration. The formulations used were (percentages octanoic acid, 1-pentanol, 1-octanol, DEP): Vibration (15.6, 8.4, 2.3 and 73.7), movement (13.6, 20.4, 45.1 and 20.9) and division (4.0, 17.9, 35.7 and 42.4). Full size image We have shown that it is possible to use a robotic system to assist in the evolution of oil droplets as models for evolvable protocells [25] . This work demonstrates that it is possible to select simple chemical systems with a desired function or trait without complete mechanistic understanding, using a system-level evolutionary approach. Not only can the platform be used to explore simple oil-droplet formulations selected for specific functions, we hope this system can be used to explore the concept of oil droplets with the ability to catalyse their own formation [26] . As a result, we hope this work will give a new direction to study how minimal information inputs, coupling chemical assemblies with algorithms, can lead to spontaneously emerging complex evolutionary systems. In summary, we believe that the platform and experimental work presented could result in a viable new perspective in the study of plausible candidates for the origin of life. In particular, this approach should allow us to explore the minimal requirements for the initiation of evolutionary dynamics. Indeed, the platform could be used to explore plausible pathways from a given chemical soup to an autonomously evolving system, perhaps stepwise to a system capable of open-ended evolution. This is because the system presented utilizes a robotic assistant as an evolutionary support system, which enables the traversal of evolutionary landscapes and the continued replication of genomic information without the need for full viability in the chemical system. While most of the characteristics of ‘life’ are wholly dependent on the robotic adjunct, in the current system, we propose that these dependencies could be removed stepwise, in serial evolutionary experiments, to move the chemical system towards full autonomy, avoiding the all-or-nothing barrier that currently plagues the study of minimal chemical replicators. It is therefore our intention to focus follow-up work towards the creation of artificial life-like assemblies, driven by a thesis that is chemically agnostic, thereby opening up investigations of new evolvable chemical systems. The chemical properties and uses of these droplet formulations will be explored in more detail in a subsequent publication. Evolutionary trajectories Statistical analyses were carried out on the evolutionary trajectory of each of the three optimization experiments. The raw fitness distributions, as a function of generation, are shown in Supplementary Fig. 14 . It is stated in the introduction that the final population of droplets, in all cases, shows enriched fitness compared with the initial populations. This analysis was performed by comparison of generation 1 with generation 21. It is common, in biological scenarios, to consider the fitter members of a population, rather than the average, since these will propagate. P values for this analysis were therefore conducted by comparing only the top half (fitness greater than the median) of each generation. This resulted in 38 individuals per generation (all three repeats were amalgamated). ANOVA was then performed with fitness as a function of generation (21 or 1) and is summarized in Supplementary Table 3 . From the results presented in Supplementary Fig. 14 , it not visually obvious whether population fitness shows improvement during the latter half of each run. To determine whether this was the case or not, the same analysis as above was repeated, but with generation 21 compared against generation 11. As can be seen in the results presented in Supplementary Table 4 , both division and vibration showed significant improvement from the halfway point to the end. Motility, however, can be considered as having been optimized after the conclusion of 11 generations. It was then questioned whether there is a significant difference in fitness variation as a function of generation. For this analysis, all generations were examined under an ANOVA, comparing continuous fitness against categorical generation number. The results are summarized in Supplementary Table 5 ; all environments showed a highly significant result. Finally, it was tested whether there was a positive dependence of fitness upon generation (that is, whether fitness increased positively with generation). Owing to the nonlinear association that was visually observed from Supplementary Fig. 14 , the Kendall correlation test was used. The results are summarized in Supplementary Table 6 ; all environments showed a highly significant result. Preparation of solutions TTAB (6.73 g, 20.0 mmol) was dissolved in distilled water ( ca 600 ml), adjusted to pH 13 with 5 M NaOH solution and made up to 1 l to give a 20-mM solution at pH 13. The oils (1-octanol, octanoic acid, dodecane, 1-pentanol and DEP; Supplementary Table 2 ) were prepared in 200 ml aliquots in reagent bottles. Each oil was dyed with 0.25 mg ml −1 Sudan III and vortexed to mix. Cleaning cycle After each experiment, acetone ( ca 3 ml) was pumped into the Petri dish to dissolve remaining oil droplets and the mixture was aspirated from the dish to the waste container. The dish was then washed with acetone (2 × 3 ml) and aqueous phase (2 × 3 ml). Less thorough cleaning cycles were often to leave trace residues, which interfered with subsequent experiments. This process is outlined in Supplementary Fig. 11 . Protocol A fully automated liquid-handling robot capable of producing droplets in a Petri dish with an aqueous subphase was constructed. The robot was based upon a RepRap 3D printer architecture with a webcam for video recording/image analysis. The droplet formulations are produced in well plates (96-well format) where each well is stirred with a magnetic stirrer bar. The droplet formulations are based upon the following reagents (1-octanol, 1-pentanol, DEP, dodecane and dilutions of octanoic acid in one of the other oils (typically 20% v/v)). The formulations were delivered from the computer control in the form of four numbers, which represented the proportion of each oil; therefore, the total summed to ‘1.0’. The total volume of the oils placed in a well was 360 μl. The specific quantity for each oil was this volume multiplied by their relative proportion. Once the mixing was completed, three experiments were conducted from the final formulation. For each experiment, 80 μl of oil were absorbed using the syringe. Of this volume, four 5-μl oil droplets are then placed in the aqueous phase (20 mM aqueous TTAB, adjusted to pH 13 with 5 M NaOH solution). These positions were consistent between experiments, with preprogrammed x–y coordinates. The needle was laid just above the aqueous phase and the droplets were released to the surface of the liquid. Once a droplet was outside the needle, the syringe was moved up to its default position. This movement broke the tension between the droplet and the needle, depositing the droplet over the aqueous phase. This process is summarized in Supplementary Fig. 10 . A video of the resulting droplet behaviour was then recorded from beneath the dish using a camera at a resolution of 640 × 480 pixels at 60 fps from below after covering the top of the Petri dish with a white background for 60 s. After the experiment, the entire contents of the dish are automatically removed and the dish is cleaned with three washes of acetone, followed by three washes of the aqueous phase. During the acetone wash, the syringe is also cleaned with acetone. After a complete generation was concluded, the evolutionary algorithm quantifies the fitness of the formulations and calculates the next set of reagent volumes. Image analysis of the droplet behaviour against the fitness function provides the next set of inputs for the evolutionary algorithm. Image processing and droplet detection The computer vision component functioned to evaluate the behaviours, exhibited by the droplets, for further analysis by the AI component. The robot used a ‘PS3 EyeToy’ as the basic sensor, to record video data from the underside of the experimental arena. To facilitate visual analysis, a white background panel was used to cover the Petri dish, to block ambient visual noise. A resolution of 640 × 480 pixels and a frame rate of 30 fps was used for video recording. The core component of the computer vision component was the library OpenCV (version 2.4.7), with SciPy used for some additional analyses. All analyses were performed using the Python bindings for OpenCV. The computer vision (CV) component consisted of multiple image-processing pipelines, one for each behaviour that was to be evaluated. Through this pipeline, droplets were identified in raw frame data ( Supplementary Fig. 8a ) and analysed for their position, size, shape and colour. Raw frame data were presented to the image-processing pipelines in the form of RGB images, as received from the camera. No prior information was input to the image analysis pipelines. Supplementary Fig. 7 outlines the complete processing pipeline. The initial step for all pipelines began with a Hough transform, used to detect the Petri dish. Once detected, an analytic arena, slightly smaller than the Petri dish, was defined. The aim of this reduction was to remove those droplets that had been caught against the edge of the dish; these droplets were considered ‘dead’. After the Hough transform, the pipeline was split into two parallel tracks. One of these tracks, aimed at long-term analysis, was based on foreground subtraction. The objective of this track was the discovery, and removal, of ambient background from the chemical components of the experiment (droplets). Because a white background was used, only the arena, with the aqueous phase present, and droplets were present. The second track was targeted at analysis of early frames and was based on a chain of image-processing operations. The objective of the image-processing track was the discovery of closed structures, which corresponded to droplets. These structures could have any shape, as long as they could be represented by a connected component. The image-processing track began with an RGB-to-grey blurring operation, applied to remove noise. This was followed by the application of the Canny edge detection algorithm, resulting in an edge map ( Supplementary Fig. 8b ). As contours may be missing pixels, a dilation operation was applied to fill these gaps ( Supplementary Fig. 8c ). This was followed by a ‘flow fill’ operation, with the origin at pixel (0,0; Supplementary Fig. 8d ). The result of this operation was the removal of any nonclosed structure. The previously calculated Hough transform was then applied to define the operational arena ( Supplementary Fig. 9a ). The next step in the pipeline was the application of a distance transform, to remove noise and to disconnect droplets that may have been artificially connected into one structure as a result of the dilation operation ( Supplementary Fig. 9b ). These final connected components were labelled using SciPy; the labels and the borders of the connected components were sent to a watershed algorithm, to recover the original size of the droplets ( Supplementary Fig. 9c ). The foreground subtraction algorithm used a mixture of Gaussians. The default OpenCV parameters were used for fitting the mixture model, with learning rate set to 0.05. The result of the mixture model was a foreground (droplets) with background information removed. The two parallel tracks resulted each in a binary image, where pixels were either ‘on’ (pixel is part of a droplet) or ‘off’ (no droplet). These two images were combined, using a boolean ‘or’ operation to give definitive droplet-only images. The contours were then discovered on this combined image ( Supplementary Fig. 9d ). With this contour map, the area, size, shape, colour and centre of the droplets could be calculated. These data were then passed on to the fitness-specific components of the image-processing pipeline. Droplet tracking Since the camera produced 30 fps, overlapping consecutive frames to track droplets over time was enough considering the size of a droplet and how much it could move between frames. Given a droplet d t in frame t, and a set of droplets D t −1 in frame t −1, a set of candidates C t −1 was built as the droplets in D t −1 whose centre was inside an area defined as a circle with 30 pixels of radius around d t . The best candidate in C t −1 was chosen as it was the nearest droplet to d t using the Euclidean distance. If there were no droplets inside this area, or all the droplets were already assigned to another droplet, this droplet was considered new. Experimental data generation and fitness functions For each experiment, a data structure describing the positions of the droplets over time was produced. These data were used in order to rate an experiment based on different factors. During this research, the behaviours analysed in this way were ‘division’, ‘movement’ and ‘directionality’. Division was defined as the number of droplets alive at the end of the experiment. We considered as viable any droplet with an area greater than 15 pixels. The experiment aimed to find droplet recipes that would divide in a controlled manner, producing viable offsprings rather than disparate fragments. Given a droplet d , its movement was defined as the Euclidean distance described by its translation between frames t and t +1. This translation was described in pixels as the fundamental units of distance. Since between a pair of frames there can be several droplets moving, the total sum of distances described by all the droplets was divided between the number of droplets, obtaining the average distance translated per droplet. Every experiment ran for 1 min, containing a few thousands of frames. The average distance per droplet was calculated for every pair of frames, its quantity summed and then divided by the total number of frames, in order to obtain the average translation described per droplet per frame. The movement-derived fitness is then given by where N is the total number of frames in the video sequence, M is the total number of droplets observed and where ( x i,t , y i,t ) are the Euclidean coordinates of droplet i on frame t . Given a droplet d in frame t , t +1, t +2, its position for each frame in the xy plane is denoted by the points A, B and C. Two vectors were defined: as and as . By directionality of a droplet it is meant the angle between and , which represents the change of direction on a droplet-moving pattern. Low values map to droplets that move in straight lines, middle values to droplets that describe curves and high values droplets that vibrate or wobble. Inverting the dot product formula: The angle is obtained: For each experiment, the angular rotation per droplet per frame was used as the directional fitness, as given by How to cite this article : Gutierrez, J. M. P. et al. Evolution of oil droplets in a chemorobotic platform. Nat. Commun. 5:5571 doi: 10.1038/ncomms6571 (2014).